Exotic non-Abelian anyons from conventional fractional quantum Hall states Non-Abelian anyons—particles whose exchange noncommutatively transforms a system’s quantum state—are widely sought for the exotic fundamental physics they harbour and for quantum computing applications. Numerous blueprints now exist for stabilizing the simplest type of non-Abelian anyon, defects binding Majorana modes, by interfacing widely available materials. Here we introduce a device fabricated from conventional fractional quantum Hall states and s -wave superconductors that supports exotic non-Abelian defects binding parafermionic zero modes, which generalize Majorana bound states. We show that these new modes can be experimentally identified (and distinguished from Majoranas) using Josephson measurements. We also provide a practical recipe for braiding parafermionic zero modes and show that they give rise to non-Abelian statistics. Interestingly, braiding in our setup produces a richer set of topologically protected operations when compared with the Majorana case. As a byproduct, we establish a new, experimentally realistic Majorana platform in weakly spin–orbit-coupled materials such as gallium arsenide. The search for non-Abelian anyons has been a major focus of both theoretical and experimental efforts in the past decade, driven largely by their potential utility for topological quantum computation [1] . Historically, the first physical system predicted to harbour such exotic quasiparticles was a fractional quantum Hall state at 5/2 filling [2] . Chiral p + ip superconductors comprise a closely related platform for non-Abelian excitations [3] , [4] . Although the existence of intrinsic p + ip superconducting materials remains an open question, Fu and Kane [5] provided a great insight by showing that one can mimic such physics by interfacing an ordinary s -wave superconductor with a topological insulator. Subsequent work distilled this architecture down to more conventional semiconductor-based setups [6] , [7] . In the above systems, non-Abelian anyons arise from Majorana zero modes bound to vortices [3] , [4] . Kitaev demonstrated that Majorana zero modes can also appear in a one-dimensional (1D) topological superconductor, and there have been several proposals applying the above ideas to 1D realizations [8] , [9] , [10] . Recent experiments have provided the first tantalizing signatures of Majorana modes in such devices [11] . Remarkably, even in networks of 1D wires Majorana zero modes generate non-Abelian statistics [12] , [13] , [14] . The aforementioned systems feature non-Abelian anyons that are not computationally universal [15] . That is, braiding operations alone cannot approximate all unitary quantum gates. Several proposals to circumvent this problem exist [16] , [17] but are either unrealistic or require non-topological operations, hence weakening the main advantage of using anyons—immunity from decoherence. Thus, whether realistic condensed matter systems can host other types of non-Abelian anyons remains an important question. Although there is some hope that certain quantum Hall plateaus may realize anyons with computationally universal braid statistics [1] , [18] , supporting experimental evidence has yet to appear. Inspired by rapid advances in the pursuit of Majorana zero modes in quantum wires, here we ask whether one can engineer a quasi-1D platform featuring more exotic non-Abelian anyons. We stress that important work by Fidkowski and Kitaev [19] appears to categorically rule out this possibility. Indeed, these authors proved that the only non-trivial zero modes supported by 1D electron systems—even with strong interactions—are Majorana fermions. We will show that this naively insurmountable restriction can be overcome by forming the 1D system out of the edge states of topologically non-trivial materials. Because the surrounding vacuum is then non-trivial, the properties of such systems are not constrained by Fidkowski and Kitaev’s classification. Our study explores devices fabricated from superconductors and conventional quantum Hall states (for example, at 1/3 filling) that appear in many materials, including gallium arsenide (GaAs) quantum wells and graphene. We show that the quantum Hall edge states in such structures support parafermionic zero modes that reflect a further fractionalization of the electronic degrees of freedom beyond that found in Majorana platforms. These modes can be experimentally probed via Josephson and tunneling measurements. Using an efficient new formalism developed here, we demonstrate that the parafermions underpin richer non-Abelian statistics than Majoranas, rendering them better candidates for quantum computation. Specifically, braiding parafermionic zero modes allows entanglement of multiple quantum information registers (qudits). These results highlight the vast potential for designing novel phases of matter using conventional materials, and open numerous experimentally relevant directions in the search for exotic non-Abelian anyons. Parafermions from a clock model To set the stage for our proposal, it is instructive to review a toy model discussed recently by Fendley [20] that supports parafermionic zero modes akin to those that we will later realize in a physical electronic system. First, we recall the well-known connection between the transverse field Ising model and a spinless p -wave superconductor: the Hamiltonians for these physically distinct systems map to one another under a non-local Jordan–Wigner transformation that trades the bosonic spin variables for fermions. Although the Ising model exhibits only conventional paramagnetic and ferromagnetic phases, the corresponding superconducting system is far more exotic. Indeed, although the paramagnetic phase of the former maps to a trivial superconducting state in the latter, the ferromagnetic phase corresponds to a topological state featuring Majorana zero modes that generate non-Abelian statistics [8] , [12] , [13] , [14] . Fendley’s insight (guided by the identification of parafermionic fields in the two-dimensional (2D) clock model [21] ) is that one can access still more exotic zero modes by implementing a non-local transformation on the generalized N -state quantum clock model [20] , Here, J ≥0 couples neighboring clock states ferromagnetically, h ≥0 is the transverse field, j labels sites of an L -site chain, and σ j and τ j are unitary operators defined on an N -state Hilbert space that satisfy . The only non-trivial commutation relation among these operators reads σ j τ j = τ j σ j e 2 πi / N . When N =2, equation (1) reduces to the familiar transverse field Ising model, though the phases realized in this special case appear also for general N . For example, with J =0, h >0, there exists a unique paramagnetic ground state with τ j =+1, whereas in the J >0, h =0 regime, an N -fold degenerate ferromagnetic ground state with σ j = e 2 πiq / N emerges ( q =1,…, N ). Consider now the non-local transformation [20] The properties of σ j and τ j dictate that these new operators satisfy , and The Methods section provides some additional useful relations. For N =2, the operators α j are self-Hermitian, anticommute and square to the identity—hence, they are Majorana fermions. At larger N , they define parafermions [20] , [21] , [22] . In these variables, the Hamiltonian becomes where h.c. is the hermitian conjugate. The phases of the clock model appear in this representation as follows. In the paramagnetic limit with J =0, parafermions dimerize as shown in Fig. 1a . Each dimer can be simultaneously diagonalized, leading to a unique, fully gapped ground state (see Methods). More interestingly, the ferromagnetic case h =0 produces the shifted dimerization shown in Fig. 1b . Again there is a bulk gap, but the ends of the chain now support unpaired zero modes α 1 and α 2 L that encode the N -fold degeneracy of the clock model’s ferromagnetic phase admits N distinct eigenvalues that do not affect the energy). At N =2, the zero mode operators α 1,2 L form the unpaired Majoranas identified by Kitaev [8] ; for N >2, they correspond to the parafermionic zero modes [20] whose physical realization is the focus of this manuscript. 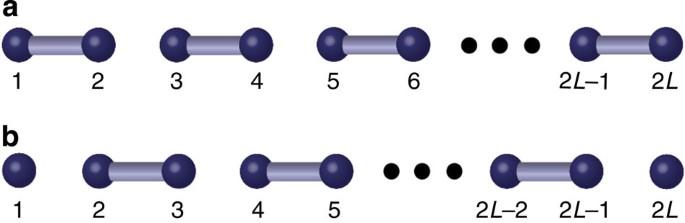Figure 1: Parafermion chain. Schematic illustration of the parafermion chain Hamiltonian in equation (4) when (a)J=0 and (b)h=0. In the latter case, the ends of the chain support unpaired parafermionic zero modes that give rise to anN-fold ground-state degeneracy. Figure 1: Parafermion chain. Schematic illustration of the parafermion chain Hamiltonian in equation (4) when ( a ) J =0 and ( b ) h =0. In the latter case, the ends of the chain support unpaired parafermionic zero modes that give rise to an N -fold ground-state degeneracy. Full size image Practical realization in 2D electron systems The Majorana zero modes supported by equation (4) when N =2 are relatively easy to engineer, as the operators α j then satisfy familiar fermionic anticommutation relations (see equation (3)). This property allows one to rewrite the N =2 Hamiltonian in terms of ordinary fermion operators c j =( α 2 j −1 + iα 2 j )/2, yielding a model for a spinless p -wave superconductor [8] that can be realized in a variety of experimental architectures [23] , [24] . However, the non-standard commutation relations obeyed by α j with N >2 makes devising experimental realizations of parafermionic zero modes substantially more difficult. Our approach is inspired by the observation that commutation relations akin to those in equation (3) do occur among physical operators in a familiar system—a fractional quantum Hall edge. For Laughlin states at filling factor ν =1/ m ( m is an odd integer), the quasiparticle operators e iφ ( x ) that create right-moving charge e / m excitations at position x along the edge obey [25] Such a system therefore provides a natural building block for a device supporting localized parafermion modes. A single quantum Hall state is insufficient for this purpose, because its edge cannot be gapped out (and, hence, one cannot localize modes of any type at the edge). Thus, we consider the geometry of Fig. 2a , where two adjacent 2D electron gases (2DEGs), each at filling ν =1/ m , produce a pair of counterpropagating edge states at their interface. These modes can acquire a gap via two different mechanisms: first, by electrons backscattering across the interface, and second, by electrons from each edge assembling into Cooper pairs. Such processes can be induced in numerous physical setups. We focus on the conceptually simplest example below but propose several viable alternatives in the Discussion. 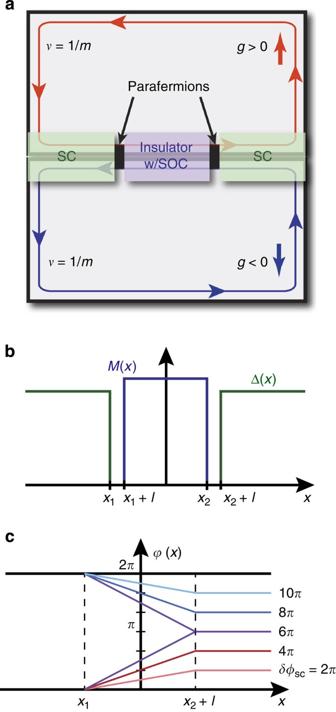Figure 2: Overview of proposed device. (a) Experimental architecture realizing parafermion zero modes. (b) Spatial profile for the electron pairing and backscattering amplitudes Δ(x) andinduced by the superconductors and insulator in (a). (c) Schematic dependence ofϕ(x) on the phase differenceδφscbetween the superconductors inain them=3 case. Asδφscwinds, the larger mismatch betweenϕ(x) on the left and right increases the energy untilδφsc=6π. Additional 2πcycles then untwistϕ(x) until the ground state is again accessed atδφsc=12π. Remarkably, this implies that the Josephson current exhibits 12πperiodicity inδφsc. Figure 2: Overview of proposed device. ( a ) Experimental architecture realizing parafermion zero modes. ( b ) Spatial profile for the electron pairing and backscattering amplitudes Δ( x ) and induced by the superconductors and insulator in ( a ). ( c ) Schematic dependence of ϕ ( x ) on the phase difference δφ sc between the superconductors in a in the m =3 case. As δφ sc winds, the larger mismatch between ϕ ( x ) on the left and right increases the energy until δφ sc =6 π . Additional 2 π cycles then untwist ϕ ( x ) until the ground state is again accessed at δφ sc =12 π . Remarkably, this implies that the Josephson current exhibits 12 π periodicity in δφ sc . Full size image To facilitate Cooper pair formation, we will assume that the 2DEGs exhibit opposite-sign g -factors, so that the red and blue edge states in Fig. 2a carry antiparallel spins. In practice, one can control the sign of the g -factor by various means [26] , [27] . The counterpropagating edge modes are then similar to those of 2D non-interacting topological insulators [28] , [29] , [30] when m =1 and fractional topological insulators [31] when m >1. This allows a pairing gap to open at the interface via the proximity effect with ordinary s -wave superconductors (green in Fig. 2a ). The spin–orbit coupling necessary for a backscattering-induced gap can arise either directly from the 2DEGs or from the insulator (purple in Fig. 2a ) that electrons traverse when crossing the interface. Domain walls separating regions gapped by these different means are particularly interesting here. We explore their properties first by considering the domain structure of Fig. 2a , assuming for simplicity that electrons backscatter across the interface only via the central insulator and form Cooper pairs elsewhere. In terms of fields φ R/L satisfying and , low-energy right- and left-moving e / m quasiparticles are created by operators that exhibit commutation relations of the form in equation (5). These properties ensure that the electron operators given by obey Fermi statistics. Below, it will prove useful to write φ R/L = ϕ ± θ ; here, ρ = ∂ x θ / π is the electron density operator while We model the interface with a Hamiltonian H = H 0 + H 1 , where [25] describes gapless counterpropagating edge modes with speed v and H 1 encodes couplings induced by the superconductors and spin–orbit-coupled insulator in Fig. 2a . For simplicity, we neglect Coulomb interactions between the edge states throughout; also, until specified otherwise, we set the superconducting phases to zero. In terms of electron operators, we have , where the profiles for the pairing and backscattering amplitudes Δ( x ) and appear in Fig. 2b . One can alternatively express H 1 using ϕ and θ variables as Similar models have been studied previously in the m =1 case, where it is well-established that each domain wall binds a single Majorana fermion [32] , [33] . We now demonstrate that for m >1, the Hamiltonian supports precisely the localized parafermion zero modes that we seek. Consider the limit where the induced pairing and backscattering terms are sufficiently strong that beneath each superconductor ϕ locks to one of the 2 m minima of the first term in equation (8), whereas under the insulator, θ pins to the minima of the second. Using the coordinates specified in Fig. 2b , one can then write , and , where and are integer-valued operators. Importantly, equation (6) yields whereas the other integer-valued operators commute. At low energies, one can focus on the intervals between x j and in Fig. 2b where Δ( x ) and simultaneously vanish, allowing both ϕ and θ to fluctuate. These regions are governed by an effective Hamiltonian subject to boundary conditions imposed by the adjacent gapped regions. As outlined in the Methods, the operators commute with H eff , and thus represent zero modes bound to the domain walls in Fig. 2 . Note that α j alters the charge by e / m ; the first term simply involves , whereas the other terms similarly add charge e / m . Apart from these modes H eff also supports excitations with a finite-size gap of order . Upon projecting out these gapped excitations, the integral in equation (11) collapses to an unimportant constant (see Methods). One then obtains the elegant expression that describe the action of the zero modes within the ground-state manifold. From equations (9) and (12), it follows that Thus, the zero modes bound to our domain walls indeed provide a physical realization of the parafermions supported by the model shown in Fig. 1 (with N =2 m ). In the present context, these modes produce a 2 m -fold ground-state degeneracy corresponding to the distinct eigenvalues of One can gain intuition for this result by noting that because , tunnels between adjacent minima of the term induced by the spin–orbit-coupled insulator. The 2 m distinct eigenstates of comprising the ground-state manifold can therefore equivalently be viewed as linear combinations of the 2 m eigenstates of characterizing the central region. In the limits studied so far, the degeneracy produced by α 1 and α 2 is exact. These modes will, however, inevitably hybridize in the more realistic situation where ϕ and θ are not perfectly pinned by the pairing and backscattering terms. Tunneling of e / m quasiparticles between the parafermions at lowest order produces a Hamiltonian Because of the gap in the region between the parafermions, the coefficient A is exponentially small in and the spacing between domain walls. Thus, the ground states remain degenerate within exponential accuracy—enabling non-local storage of a 2 m -state topological qudit. As occurs with Majorana fermions [8] , [5] , the parafermions in our system mediate spectacular signatures in Josephson measurements. To illustrate this, let us revisit the setup of Fig. 2a in the limit where ϕ and θ are pinned by the superconductors and insulator. Suppose that after initializing the system into one of the resulting 2 m ground states, the backscattering amplitude adiabatically decreases to zero, so that the parafermions strongly hybridize between the superconductors. We assume that the central region of Fig. 2a remains gapped by finite-size effects even when . Our goal is now to study the Josephson current flowing across the junction when the superconducting phase on the left side remains zero, whereas the phase on the right, δφ sc , varies. The Hamiltonian describing this configuration is , where H 0 is again given in equation (7), whereas Suppose first that when δφ sc =0, we begin in a ground state with and . Upon smoothly increasing δφ sc to 2 π , our initial state evolves such that ϕ > = δφ sc /2 m to minimize the second term in equation (15). Crucially, this cycle raises the system’s energy because of the mismatch between ϕ < and ϕ > ; the resulting twist of ϕ ( x ) between the superconductors costs energy due to the ( ∂ x ϕ ) [2] term in H 0 . The system returns to its original state only after δϕ sc winds by 4 πm , after which one obtains a value φ > =2 π that is physically equivalent to our initial value of 0. Figure 2c shows the simplest non-trivial case with m =3. The Josephson current I 0 ( δφ sc ) d〈 H 〉/d δφ sc follows from the energy and, hence, also admits 4 πm periodicity. (See Supplementary Methods for a more quantitative treatment.) Interestingly, the current–phase relation depends sensitively on the initial state. Consider the more general situation where, before fusing the parafermions across the junction, we prepare the system into a ground-state characterized by , for some integer δn . One can generalize the above analysis to show that the current becomes I δn ( δφ sc )= I 0 ( δφ sc +2 πδn ), which differentiates all physically distinct values of δn . Thus, the 4 πm -periodic Josephson effect both provides a definitive signature of the parafermions in our setup and enables readout of the quantum information they store [5] . Parafermion braiding The results thus far extend straightforwardly to setups exhibiting arbitrarily many domain walls separating pairing- and backscattering-gapped regions. domain walls localize parafermion zero modes (numbered from left to right) that obey equation (13) and produce degenerate ground states. Next, we show that these modes generate non-Abelian statistics and allow one to perform a richer set of topologically protected operations on the ground-state manifold than are available in the Majorana case. As a first step, we introduce a practical recipe for transporting domain walls and a geometry that permits their meaningful exchange. To mobilize the domain walls, we turn to the setup of Fig. 3a . Here the 2DEGs couple to a superconductor and spin–orbit-coupled insulator throughout the interface, whereas gates below control the potential along the edges. The Hamiltonian describing the interface is then H = H 0 + H 1 + H μ , with H 0,1 given by equations (7) and (8) but now with uniform and Δ. The induced potential μ ( x ) generates the third term, H μ =−∫d xμ ( x ) ∂ x θ / π (recall that the electron density is ρ = ∂ x θ / π ). We assume , so that when μ ( x )=0, a gap arises from inter-edge tunneling. Suppose that starting from this regime we adjust the gates to raise μ uniformly. Shifting eliminates the resulting potential term H μ but, crucially, also sends . The spatial oscillations render the backscattering term ineffective, so that the pairing energy Δ can then dominate. More physically, gating changes the momentum carried by low-energy quasiparticles, which affects inter-edge tunneling ( ) but not Cooper pairing ( ψ R ψ L ). The gates in Fig. 3a thereby allow one to dynamically control the nature of the gap in each region, and hence manipulate domain walls in real time. 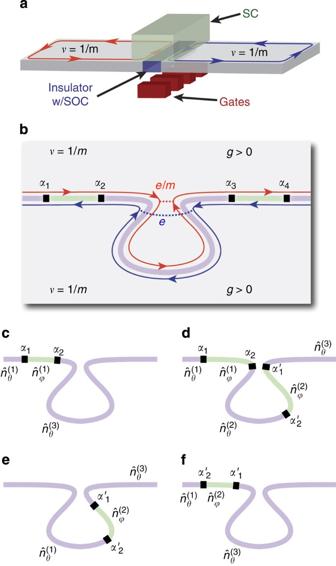Figure 3: Transport and braiding. (a) Setup allowing adiabatic domain wall transport via gating. (b) Sack-like geometry that permits braiding of domain walls between tunneling-gapped (purple) and pairing-gapped (green) regions. Parafermionic zero modes are denoted byαj. Clockwise exchange of domain walls bindingα1andα2proceeds as outlined (c–f), whereanddescribe the pinnedϕandθfields in a given region. Figure 3: Transport and braiding. ( a ) Setup allowing adiabatic domain wall transport via gating. ( b ) Sack-like geometry that permits braiding of domain walls between tunneling-gapped (purple) and pairing-gapped (green) regions. Parafermionic zero modes are denoted by α j . Clockwise exchange of domain walls binding α 1 and α 2 proceeds as outlined ( c – f ), where and describe the pinned ϕ and θ fields in a given region. Full size image Let us now deform the interface into the geometry sketched in Fig. 3b , where gates are tuned to localize parafermions α 1,…,4 . This setup permits exchange of any pair of domain walls shown. We will analyze the adiabatic clockwise braid of the domain walls binding α 1 and α 2 as outlined in Fig. 3c–f ; other exchanges can be understood similarly. In the figures, and denote integer operators that describe the pinned ϕ and θ fields in a given region. Equation (6) implies that for j ≥ k , while for j < k , the operators commute. Because we are concerned here only with the ground-state sector, it suffices to express , , and similarly for α ′ 1,2 . In the first step, (c)→(d), the right domain wall moves into the sack. We model this process with a Hamiltonian The t ′ term above represents charge e / m tunneling between the domain walls binding and in Fig. 3d . Similarly, t reflects e / m tunneling between the inner (red) edge states at the constriction in Fig. 3b , with β a system-dependent phase. Tunneling can also occur between the outer (blue) edge states. However, because the barrier between the 2DEGS does not support fractionalized excitations, only electrons can tunnel between these edges. Electron tunneling has no effect on our conclusions and shall henceforth be neglected. For details see Supplementary Methods . The configuration in Fig. 3c can be described by H c→d with t =0 and t ′≠0; and then hybridize while α 1,2 comprise our initial parafermionic zero modes. We then pull and apart (thus reducing t ′) while simultaneously increasing the coupling across the constriction ( t >0), arriving at Fig. 3d . Throughout this process, α 1 remains a zero mode. However, the zero mode initially given by α 2 evolves nontrivially. In principle, one can track this evolution by explicitly solving H c→d for general t and t ′—a cumbersome task even for Majoranas [12] . Here we introduce a new approach that utilizes conserved quantities to obtain the result far more efficiently. First, we observe that commutes with H c→d for any choice of parameters and hence is conserved. This should be expected on physical grounds: were and to change throughout this process, zero modes well outside of the sack (for example, α 1 ) would be affected as well. At the beginning of this step t ′ pins . Consequently, χ projects onto the initial form of the zero mode of interest, χ → α 2 . Upon completing this step, t instead imposes the energy-minimizing condition for some β -dependent integer k . Because χ is conserved, projecting onto the ground-state manifold yields the properly evolved zero mode: . Notice that this zero mode does not localize to the transported domain wall, except in the Majorana case where . Next, we transport the domain wall binding α 1 to arrive at Fig. 3e . This process can be similarly modeled by where the parameters change from t ≠0, t ′′=0 at the start of this step to t =0, t ′′≠0 at the end. In this case, the operator identified above remains a zero mode throughout, whereas now the zero mode initially given by α 1 evolves. Proceeding as above, we define , which generically commutes with H d → e and initially projects (using equation (17)) to α 1 . When the domain wall moves into the sack t ′′ pins . The zero mode formerly described by α 1 thus evolves to at the end of this step. During the final step of the exchange, where the domain walls are transported to the configuration in Fig. 3f , both zero modes evolve trivially. Let U 12 be the operator implementing the exchange. Comparing Fig. 3c to 3f , one finds that the parafermions transform as Note that the analogue of parity in the Majorana case—is preserved here. We would now like to understand how the braid transforms the 2 m degenerate ground states. Assuming α 1,2 are the only zero modes, we denote these states by | q 〉 where . Equation (19) implies that (up to an overall phase) With additional domain walls, non-Abelian operations become available. For example, if U 23 implements a clockwise exchange of the domain walls binding α 2 and α 3 in Fig. 3c , then , whereas . Remarkably, braiding parafermionic zero modes brings one closer to computational universality than braiding Majoranas. Indeed, we show in the Supplementary Methods that exchanging two pairs of parafermions produces a controlled phase gate CP =( U 23 U 12 U 34 U 23 ) [2] that can entangle the state of the pair α 1 , α 2 with that of the pair α 3 , α 4 . Up to an overall phase, this operation yields where q and q ′ label the eigenvalues of and , respectively. Such an entangling gate is unavailable through braiding of Majorana modes, where m =1. In this paper, we introduced an experimental setup employing conventional quantum Hall edge states to localize exotic non-Abelian anyons. In the integer quantum Hall case ( m =1), our proposal paves the way towards realizing Majorana wires in weakly spin–orbit-coupled systems such as GaAs. The fractional case ( m >1) constitutes a much more important advance, as here our device provides a route to engineering networks of parafermion zero modes that can be moved along 1D channels. Although we focused on a setup with the virtue of conceptual clarity, numerous simplifications of the architecture introduced here are possible. The insulators in Figs 2 and 3 can be dispensed with entirely, as spin–orbit coupling can instead arise from the 2DEGs themselves. One also need not employ opposite-sign g -factors to generate Cooper pairing [34] ; a proximity effect can still appear if spin is not conserved in either the 2DEGs or the parent s -wave superconductors [35] or if one employs superconductors with a triplet component [36] . Graphene provides a particularly promising 2DEG, given the experimental evidence of superconducting proximity effect, even in the quantum Hall regime [37] . Yet another variation could employ bent quantum Hall systems pioneered by Grayson et al . [38] , [39] , which could provide an effective geometry for obtaining well-coupled Laughlin edge states. We have shown that parafermion zero modes can be identified—and distinguished from Majoranas—via Josephson measurements. Tunneling experiments may provide a less definitive, though perhaps easier, probe. Indeed, if α j represents a parafermion zero mode then is a Majorana operator that can couple to electrons from a lead; thus, parafermions give rise to the same quantized zero bias anomaly as Majoranas [40] . Experimental verification may also be possible using resonant tunneling of e / m charges in a setting where a parafermion mode localizes inside a quantum Hall point contact (with tunneling charge detectable by, for example, noise measurements [41] ). In the future, it will be interesting to address whether one can create even more exotic non-Abelian anyons (for example, Fibonacci) using other fractional quantum Hall states beyond the Laughlin series considered here. Another worthwhile extension of our work would be to explore three-dimensional fractional topological insulators with proximity-induced superconductivity to generalize Fu and Kane’s proposal [5] and search for realizations of novel models such as that of You and Wen [42] . And finally, an important question for future applications is whether one can utilize parafermions to more readily achieve universal quantum computation. To that end, we note that braiding of Majoranas must be supplemented by two additional gates to achieve universality [1] . The first is a single-qubit phase gate, which together with braid transformations completes the set of single-qubit unitary operations. The second is a multi-qubit entangling gate that may be obtained, for example, by measuring the topological charge of four Majoranas via interference. Although the first type of gate remains absent in the parafermion case, the CP braid described above eliminates the need for interferometry by generating entanglement through braiding alone. This gate, combined with arbitrary single-qudit operations, is universal for quantum computation. We leave to future work an investigation of how such single-qudit operations might be realistically performed. Properties of parafermionic operators Here we will enumerate several useful properties of parafermion operators that follow from the definitions provided in the main text. Because and , these operators are unitary and exhibit eigenvalues of the form e 2 πiq / N for integral q . The second equation together with the commutation relations in equation (3) imply that Moving past , therefore, produces the opposite phase factor compared with moving past . Consequently, we obtain the following commutation relations, which further imply that so long as neither k nor l lie between i and j . Equations (23) and (24) demonstrate that as claimed in our discussion of the 1D clock model, one can indeed simultaneously diagonalize each of the dimers sketched in Fig. 1 , as well as the combination of zero-mode operators in Fig. 1b . To deduce the allowed eigenvalues, we note that one can show from the properties above that which constrains the eigenvalues of to the form , where q is an integer. In the quantum clock model context, the eigenvalues of the relevant dimer operators can alternatively be found using the relations that arise from the non-local transformation specified in equation (2). Equations (26) yield the same eigenvalue spectrum for the operators on the left-hand side as noted above, because τ j and σ j both exhibit non-degenerate eigenvalues e 2 πiq / N for q =1,…, N . Finally, we consider the case where α 1 and α 2 L represent zero modes and deduce the action of these operators on the ground-state manifold. Let | q 〉 be a ground state satisfying . Using the parafermion commutation relations one can show that for either j =1 or 2 L . This equation implies that and , where the proportionality constants have unit magnitude. One can always fix the relative phases of the ground states such that With this convention, α 2 L then acts as follows: Solution for localized parafermion zero modes Here we provide a detailed derivation of the localized parafermion zero-mode operators quoted in the main text (equation (11)). Consider again the static domain structure of Fig. 2a . As in the main text, we will assume that the Cooper pairing and inter-edge tunnelling terms induced at the interface are sufficiently strong that ϕ ( x ) is pinned beneath the superconductors, whereas θ ( x ) is pinned beneath the spin–orbit-coupled insulator. In the black regions of width in Fig. 2a , however, both fields can fluctuate because the pairing and tunnelling terms simultaneously vanish there. Our objective is to now understand the low-energy properties of these regions, which will eventually lead us to the parafermionic zero-mode operators of interest. For clarity, we examine each domain wall separately, beginning with the one on the left. At low energies, this domain wall is governed by an effective Hamiltonian Minimizing the energy of the adjacent gapped regions requires that these fields also satisfy boundary conditions and for integer-valued operators and (recall equation (8)). Note that and commute because according to equation (6). Equation (30) can be diagonalized by expanding the ϕ and θ fields as where and a k correspond to conventional bosonic operators satisfying . This decomposition simultaneously preserves the commutation relations among ϕ ( x ) and θ ( x ′) and encodes the boundary conditions specified above. Inserting equation (31) into the Hamiltonian yields Thus, we see that the a k bosons exhibit a finite-size gap inversely proportional to . This does not, however, necessarily imply that the domain wall admits only gapped excitations. We will now demonstrate that, because the operators and both commute with the Hamiltonian, the domain wall supports zero modes that can be constructed from local operators present in our edge theory. To do so, it is convenient to work with chiral fields ϕ R/L instead of ϕ and θ . From equation (31), we have which yields the useful relations One can employ equations (32) and (34) to show, with the aid of various commutator identities and some algebra, that As the right-hand side is a total derivative, the above equation integrates to Finally, equations (35) and (37) allow one to demonstrate that the operator commutes with the Hamiltonian and therefore represents a zero mode of the system. Several points are worth emphasizing here. First, α 1 is constructed purely from local e / m quasiparticle operators , and thus represents a physical zero mode bound to the domain wall. To see this explicitly, observe that and always appear in α 1 via and . Second, the expression for the zero mode quoted above is not unique; one can always multiply α 1 by allowed operators (such as H or that also commute with the Hamiltonian. This freedom—which is a generic feature of zero-mode operators—is, however, inconsequential for our purposes. We are concerned here only with the physics of the ground-state manifold and in operators that cycle the system among the various ground states. For this purpose, the form of α 1 above suffices. Third, note from equation (34) that the integrand in equation (38) involves only bosonic operators (and not or ). This makes the projection of α 1 into the ground-state manifold with very simple; upon discarding an overall constant one obtains the result quoted in the main text. The right domain wall in Fig. 2a can be analyzed very similarly. Here the effective low-energy Hamiltonian is given by where now the fields satisfy boundary conditions and . Because the left and right domain walls of Fig. 2a are bridged by a single spin–orbit-coupled insulator, and θ ( x 2 ) must be pinned to identical values. Thus, is the same integer-valued operator that we introduced above. However, ϕ ( x 1 ) and are pinned by different superconductors, which necessitates the introduction of distinct integer-valued operators . Importantly, in this geometry and no longer commute because equation (6) yields . Given our new boundary conditions, the appropriate decomposition for ϕ and θ reads with and as before. With this expansion, our low-energy Hamiltonian once again takes the form in equation (32). One can then follow the steps outlined above (taking care to enforce the non-trivial commutation relations between and ) to show that the right domain wall binds a zero mode described by an operator Projecting onto the ground-state manifold yields, up to a constant, How to cite this article : Clarke, D.J. et al . Exotic non-Abelian anyons from conventional fractional quantum Hall states. Nat. Commun . 4:1348 doi: 10.1038/ncomms2340 (2013).